Resonant bonding leads to low lattice thermal conductivity Understanding the lattice dynamics and low thermal conductivities of IV–VI, V 2 –VI 3 and V materials is critical to the development of better thermoelectric and phase-change materials. Here we provide a link between chemical bonding and low thermal conductivity. Our first-principles calculations reveal that long-ranged interaction along the 〈100〉 direction of the rocksalt structure exist in lead chalcogenides, SnTe, Bi 2 Te 3 , Bi and Sb due to the resonant bonding that is common to all of them. This long-ranged interaction in lead chalcogenides and SnTe cause optical phonon softening, strong anharmonic scattering and large phase space for three-phonon scattering processes, which explain why rocksalt IV–VI compounds have much lower thermal conductivities than zincblende III–V compounds. The new insights on the relationship between resonant bonding and low thermal conductivity will help in the development of better thermoelectric and phase change materials. Most good thermoelectric and phase-change materials are found in group IV–VI, V 2 –VI 3 and V materials. For example, PbTe, Bi 2 Te 3 and Bi 1−x Sb x have been the best thermoelectric materials in the intermediate, room and low-temperature ranges, respectively [1] , [2] , [3] , [4] . Alloys of GeTe and Sb 2 Te 3 (GST) have been the most popular materials for optical storage technologies such as compact disc and phase-change random access memory [5] , [6] . These materials all have low thermal conductivity, which is crucial for thermoelectric and phase-change memory applications. Usually, group IV–VI, V 2 –VI 3 and V materials have low thermal conductivity. This becomes particularly obvious when IV–VI materials are compared with III–V compounds. For example, the thermal conductivity of SnTe is only 4 W/m-K while that of InSb, adjacent to SnTe in the periodic table, is 16 W/m-K at room temperature [7] , [8] . The low thermal conductivities of rocksalt IV–VI materials (hereafter IV–VI materials) compared with those of zincblende III–V materials (hereafter III–V materials) have been attributed to their differences in the crystal structure. While III–V materials have tetrahedral bonding, many IV–VI materials have octahedral bonding. The bond length is usually longer in octahedral structures than in tetrahedral structures, resulting in weaker bonding and lower thermal conductivity [9] . Our first-principles calculations show that there are more reasons for the low thermal conductivities of IV–VI materials than that discussed above. To compare the thermal conductivities of many different III–V and IV–VI materials, we normalized their thermal conductivities by harmonic properties using the formula suggested by Slack [10] . The formula gives reasonable predictions for many materials with zincblende and rocksalt structures [11] . According to the formula, thermal conductivity is given by where B is a numerical coefficient, is the average mass of the basis atoms, n is the number of phonon branches and γ is the Grüneisen parameter. The average volume per atom is denoted by δ 3 , and θ is the acoustic Debye temperature. Here, harmonic properties include , θ and δ ; these three properties determine the average group velocities of acoustic phonons and they reflect the bonding stiffness. In Fig. 1 , we plot the thermal conductivities, κ , of IV–VI and III–V materials normalized by the harmonic properties, , as a function of the mass ratio of the basis atoms. There are two distinct differences between the thermal conductivities of IV–VI and III–V materials: (1) overall, IV–VI compounds still have much lower thermal conductivities than III–V compounds even after normalization, and (2) the thermal conductivity difference between IV–VI and III–V materials is amplified when the mass ratio is small. 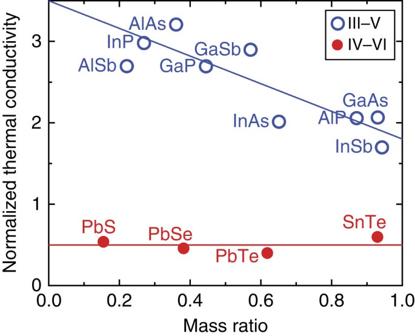Figure 1: Normalized thermal conductivities of binary III–V and IV–VI compounds at 300 K. The solid lines are for an eye guide. Figure 1: Normalized thermal conductivities of binary III–V and IV–VI compounds at 300 K. The solid lines are for an eye guide. Full size image In this work, we present an unusual behaviour in the lattice dynamics of IV–VI, V 2 –VI 3 and V materials and the origin of the two aforementioned differences in the thermal conductivities of III–V and IV–VI compounds. We first show that seemingly different IV–VI, V 2 –VI 3 and V materials commonly have long-ranged interactions along the 〈100〉 direction of rocksalt as a result of the resonant bonding. Then, we infer that the significant long-ranged interaction in IV–VI materials play a key role in their low thermal conductivities. Resonant bonding in IV–VI, V 2 –VI 3 and V materials Resonant bonding can be understood as resonance or hybridization between different electronic configurations: three valence p -electrons alternate their occupancy of six available covalent bonds that exist between a given atom and its octahedral neighbours [12] . For example, in PbTe, sp -hybridization is small and the s -band is lower than the p -band by 1.5 eV (ref. 13 ). Therefore, we can consider only p -electrons for valence states and each atom has three valence electrons on average. Given PbTe’s octahedral structure and its three valence electrons per atom, the choice of bond occupation is not unique. This leads to hybridization between all the possible choices for the three electrons forming the six bonds. This description of resonant bonding is based on IV–VI compounds and their isoelectronic V elements for simplicity, but the resonant bonding exists in even more complicated materials such as V 2 –VI 3 and many alloys of IV–VI and V 2 –VI 3 materials [14] . In general, the unsaturated covalent bonding by p -electrons with rocksalt-like crystal structures can be regarded as resonant bonding [15] . Materials with resonant bonding have several features. First, because of their coordination number of six, they have rocksalt-like crystal structures. Many IV–VI, V 2 –VI 3 and V compounds have rocksalt-like crystal structures, as shown in Fig. 2 . In addition, these materials have very weak sp -hybridization and the s -bands are well below the p -bands. Several past works show that PbTe, Bi 2 Te 3 and Bi satisfy this condition [13] , [16] , [17] and our calculations using density functional theory also present weak sp -hybridization in these materials (see Supplementary Note 1 ; Supplementary Figs 1–7 ). One very important feature of resonant bonding is that the electron density distribution is highly delocalized. As a result, the materials in this group have large electronic polarizability, dielectric constants and Born charges [18] , [19] . For example, the dielectric constants of PbTe and Bi 2 Te 3 (||) are 33 and 50, respectively, while for Si the value is 11.76 (refs 20 , 21 , 22 ). In a similar way, certain electronic properties of thermoelectric and phase-change materials have also been explained by invoking resonant bonding [12] , [15] . Matsunaga et al . [23] used experimental observations of low frequency of transverse optical (TO) phonons, so-called soft TO mode (a feature that is clear in the phonon dispersion to be shown later), to make a connection between resonant bonding and the small differences in the thermal conductivities of crystalline and amorphous phases of GST. Here, from first-principles, we provide a detailed lattice dynamics-based link between resonant bonding and the soft TO modes and low thermal conductivities of a wide range of materials. 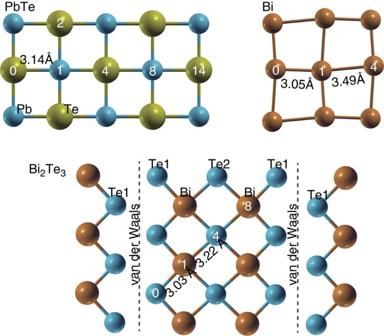Figure 2: Rocksalt-like crystal structures of PbTe, Bi2Te3and Bi. The number on each atom indicates the shell number. Bi2Te3, Bi and Sb have distorted rocksalt structures and have different numbers for shells than the exact rocksalt case. The numbers on the Bi2Te3and Bi atoms indicate the equivalent shell numbers as for a rocksalt structure in the absence of lattice distortion. Figure 2: Rocksalt-like crystal structures of PbTe, Bi 2 Te 3 and Bi. The number on each atom indicates the shell number. Bi 2 Te 3 , Bi and Sb have distorted rocksalt structures and have different numbers for shells than the exact rocksalt case. The numbers on the Bi 2 Te 3 and Bi atoms indicate the equivalent shell numbers as for a rocksalt structure in the absence of lattice distortion. Full size image Long-ranged interaction due to the resonant bonding We calculated the harmonic force constants in typical IV–VI, V 2 –VI 3 and V materials using first-principles density functional theory and found that a common feature among these compounds is the presence of long-ranged interactions along the 〈100〉 direction of rocksalt structure. To compare these different materials regardless of crystal structures and bonding stiffness, traces of interatomic force constant (IFC) tensors are normalized by the trace values of the self-interacting IFC tensor (see Supplementary Note 2 for details). From Fig. 3a , fourth-nearest neighbours, separated by 6 Å (for example, Pb-Pb and Te-Te), have interactions which are comparable to those of first-nearest neighbours, spaced 3 Å apart, and are much stronger than second- and third-nearest neighbour interactions. In addition, eighth-nearest neighbours, separated by 9 Å, have even positive force constants, giving them the behaviour of ‘anti-springs’. Fourteenth-nearest neighbours, separated by 12 Å, also have non-negligible force constants. The force constants at the fourteenth-nearest neighbours are clearly distinguished from other force constants nearby when using finer q mesh in the electron response calculation to capture the long-ranged interaction more accurately. These first-, fourth-, eighth- and fourteenth-nearest neighbours form a chain along the 〈100〉 direction in rocksalt structures, as shown in Fig. 2 . Other rocksalt IV–VI materials, such as PbSe, PbS and SnTe, exhibit very similar behaviours. These behaviours were not captured by earlier works on the lattice dynamics of PbTe and PbS within the shell model [24] , [25] . To compare lead chalcogenides and SnTe with other materials, in Fig. 3b we show that the IFCs of NaCl and InSb decrease with distance. NaCl and InSb are chosen as prototypes of ionic and sp -hybridized covalent bonding materials, respectively. The long-ranged interactions along the 〈100〉 direction in NaCl are much smaller compared with those in PbTe. In the case of InSb, interactions besides for first-nearest neighbour ones are negligible. 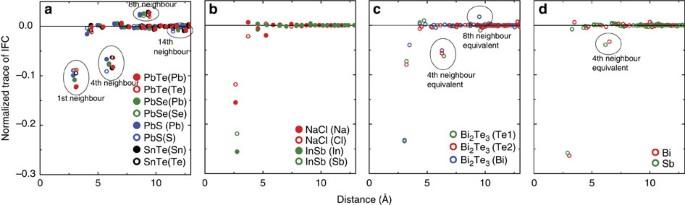Figure 3: Normalized trace of interatomic force constant tensors versus atomic distances. (a) Lead chalcogenides and SnTe (group IV–VI), (b) NaCl and InSb, (c) Bi2Te3(group V2–VI3) and (d) Bi and Sb (group V). The element in the parenthesis indicates the interaction between the corresponding atom and other atoms. For example, ‘PbTe(Pb)’ means interaction between Pb and other atoms in PbTe. Figure 3: Normalized trace of interatomic force constant tensors versus atomic distances. ( a ) Lead chalcogenides and SnTe (group IV–VI), ( b ) NaCl and InSb, ( c ) Bi 2 Te 3 (group V 2 –VI 3 ) and ( d ) Bi and Sb (group V). The element in the parenthesis indicates the interaction between the corresponding atom and other atoms. For example, ‘PbTe(Pb)’ means interaction between Pb and other atoms in PbTe. Full size image We need to point out that the long-ranged interactions we observe are different from long-ranged Coulomb interaction, which cannot explain why fourth-nearest neighbour interactions are stronger than second- or third-nearest neighbour interactions. The long-ranged and non-monotonically decreasing interaction is due to the long-ranged electronic polarizability (see Supplementary Note 3 for details). In Fig. 4a,b , we compare electron density distribution at ground state of PbTe and NaCl. From the ground-state electron density distribution, it is clear that PbTe has largely delocalized electron density distribution due to the resonant bonding, but electrons in NaCl are highly localized due to the ionic bonding. In Fig. 4e , electron polarization in NaCl is short ranged and electrons surrounding the fourth-nearest neighbours are not perturbed much. However, electron polarization in PbTe in Fig. 4f is long ranged and reaches the fourth-nearest neighbour. The electron density distribution surrounding the fourth-nearest neighbours is largely disturbed by the displacement of the center atom. 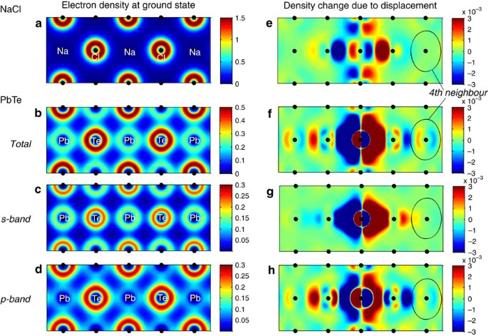Figure 4: Electron density distribution and polarization in NaCl and PbTe. (a–d) Electron density distribution at ground state. (e–h) Electron density distribution change by the displacement of the center atom. The plot is on (100) plane and each black dot represents an atom. The unit is Å−3. Figure 4: Electron density distribution and polarization in NaCl and PbTe. ( a – d ) Electron density distribution at ground state. ( e – h ) Electron density distribution change by the displacement of the center atom. The plot is on (100) plane and each black dot represents an atom. The unit is Å −3 . Full size image The long-ranged polarization in PbTe can be explained by the resonant bonding. In resonant bonding, if one atom is displaced along the +x direction, it perturbs the p x orbital of the adjacent atom. In other words, the bonding electrons on the −x side of the adjacent atom easily move to the +x side since both sides are in the same p x orbital [26] . This perturbation can persist over long ranges owing to the large electronic polarizability and the collinear bonding in resonant bonding materials. The band-by-band electron polarization analysis in Fig. 4 confirms that the long-ranged polarization is owing to resonantly occupied p -electrons. PbTe has very weak sp- hybridization and we plot the electronic polarization for s -band and p -band electrons separately in Fig. 4f–h . From Fig. 4g , the polarization of s -electron is short ranged and does not reach the fourth-nearest neighbour. However, the p -electron distribution in Fig. 4h exhibits the long-ranged polarization. This analysis shows that the easily polarized electrons in PbTe are resonantly occupied p -electrons, rather than lone pair Pb s electrons suggested in recent work [27] . The resonant bonding picture discussed above also applies to V 2 –VI 3 (Bi 2 Te 3 ) and V (Bi and Sb) materials. Bi 2 Te 3 has a rhombohedral structure that can be understood as a deformed rocksalt structure with layer spacing as shown in Fig. 2 . This rocksalt-like structure contains five resonantly bonded layers of atoms (Te1–Bi–Te2–Bi–Te1), and is separated from the next quintuple layer by weak Te1–Te1 van der Waals interactions. The structural deviation from the exact rocksalt structure within the quintuple layer is small. The lengths of the strongest bond (Te1–Bi), 3.03 Å, and that of the second-strongest bond (Bi–Te2), 3.22 Å, are similar. In addition, the angles of Te1–Bi–Te2 and Bi–Te2–Bi are 174.6° and 180°, respectively, making them similar to the rocksalt structure since the rocksalt has an angle of 180° exactly. Owing to this small structural distortion, the resonant bonding exists in a weakened form. As shown in Fig. 3c , the IFCs of Bi 2 Te 3 show a behaviour similar to that of lead chalcogenides, but the long-ranged interactions are weakened owing to the structural distortions, resulting in weakened resonant bonding. Bi–Bi and Te1–Te2, both spaced about 6 Å apart, have interactions that are equivalent to the fourth-nearest neighbour interactions in an exact rocksalt structure, and are less significant compared with the PbTe case. The interactions of Bi–Te1 (at a distance of 9 Å) separated by Te2–Bi, which are equivalent to the eighth-nearest neighbour interactions in PbTe, also have positive force constants, but their magnitudes are smaller than those of the PbTe case. However, it is noticeable that the force constants of Te2 atoms are very similar to those of the Te atom in PbTe, as predicted in previous work [19] . This is because the resonant bonding around the Te2 atom is well maintained: the Bi–Te2 and Te2–Bi bond lengths are same and they make an angle of 180°, as shown above. Another noticeable observation in Bi 2 Te 3 is that there is no long-ranged interaction between atoms separated by Te1–Te1. It is well known that Te1–Te1 has van der Waals type of bonding owing to the induced dipole–dipole interaction [16] , prohibiting the long-ranged interaction by the long-ranged electron polarization shown in Fig. 4 . Pure Bi and Sb have rhombohedral crystal structures that are Peierls distortions of simple cubic structure [28] . With the two basis atoms, the structure can be understood as a rocksalt structure stretched along the 〈111〉 direction. Because of the distortion, the six first-nearest neighbours in the rocksalt structure become three first-nearest neighbours and three second-nearest neighbours. The distances between the first- and the second-nearest neighbours are 3.05 Å and 3.49 Å, respectively. Considering that the distances between the first- and the second-nearest neighbours are 3.03 Å and 3.22 Å, respectively, in Bi 2 Te 3 , the distortion from the rocksalt structure is larger in Bi and Sb than in Bi 2 Te 3 . Therefore, the resonant bonding is further weakened in Bi and Sb and this is clearly visible in the electron density distributions of PbTe and Bi ( Supplementary Note 4 ; Supplementary Fig. 8 ). This structural distortion further weakens the long-ranged interactions, as shown in Fig. 3d . However, the ninth-nearest neighbours, separated by 6 Å, have interactions that correspond to the fourth-nearest neighbour interactions in rocksalt and are thus significant. Effects of long-ranged interaction on thermal conductivity The long-ranged interaction along the 〈100〉 direction is related to the existence of a soft TO mode. This directional long-ranged interaction was also predicted and considered as a main reason for the ferroelectric behaviour in perovskite BaTiO 3 and PbTiO 3 (ref. 29 ). We used a one-dimensional (1D) lattice chain model to explicitly show that the long-ranged interaction causes the softening of the TO mode (see Supplementary Note 5 for details). In Fig. 5a , as the second- and third-nearest neighbour interactions in the 1D chain (equivalent to fourth- and eighth-nearest neighbour interactions in rocksalt) increased, the zone center TO phonon frequency decreased. The pronounced softening of the TO modes in IV–VI materials, shown in Fig. 5b , is consistent with this 1D model. To further confirm that the long-ranged interactions along 〈100〉 are the main reason for the near-ferroelectric behaviour, phonon dispersion is calculated for fictitious PbTe without the fourth- and eighth-nearest neighbour interactions. The TO mode in the fictitious PbTe is not softened as shown in Fig. 5b . By comparison, Bi 2 Te 3 , Bi and Sb have weakened long-ranged interactions owing to distortion of the structure, and their TO modes are not as soft as those of IV–VI materials ( Fig. 5c,d ). 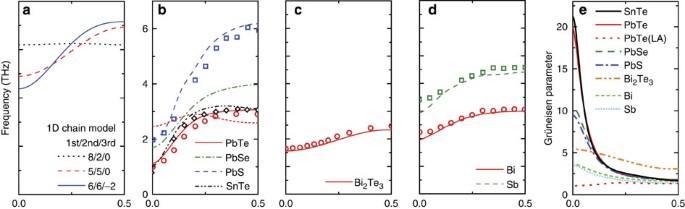Figure 5: Near-ferroelectric behaviour due to resonant bonding. (a) Optical phonon dispersion in a model 1D atomic chain, showing the softening of the optical phonons due to the long-ranged interactions. Three numbers in the legend represent relative interaction strengths of first-, second- and third-nearest neighbours in the 1D chain. (b–d) Soft TO phonon modes along the trigonal direction for lead chalcogenides, SnTe, Bi2Te3, and Bi and Sb, respectively, calculated based on first-principles. Lines and circles are calculation and experimental data, respectively. The experimental data are from refs19,24,25,49,50,51. The red dotted line inbis after removing the fourth-, eighth- and fourteenth-nearest neighbours interactions in PbTe, which does not show the soft TO mode. (b–d) are plotted in the same scale of theyaxis. (e) Calculated mode Grüneisen parameters of TO mode, showing strongly anharmonic behaviour of TO phonons of lead chalcogenides and SnTe. The red dotted line indicates Grüneisen parameters of the longitudinal acoustic mode in PbTe for comparison. Figure 5: Near-ferroelectric behaviour due to resonant bonding. ( a ) Optical phonon dispersion in a model 1D atomic chain, showing the softening of the optical phonons due to the long-ranged interactions. Three numbers in the legend represent relative interaction strengths of first-, second- and third-nearest neighbours in the 1D chain. ( b – d ) Soft TO phonon modes along the trigonal direction for lead chalcogenides, SnTe, Bi 2 Te 3 , and Bi and Sb, respectively, calculated based on first-principles. Lines and circles are calculation and experimental data, respectively. The experimental data are from refs 19 , 24 , 25 , 49 , 50 , 51 . The red dotted line in b is after removing the fourth-, eighth- and fourteenth-nearest neighbours interactions in PbTe, which does not show the soft TO mode. ( b – d ) are plotted in the same scale of the y axis. ( e ) Calculated mode Grüneisen parameters of TO mode, showing strongly anharmonic behaviour of TO phonons of lead chalcogenides and SnTe. The red dotted line indicates Grüneisen parameters of the longitudinal acoustic mode in PbTe for comparison. Full size image The TO phonon softening leads to strong anharmonicity and phonon scattering by the TO modes [30] . To show the anharmonicity of the modes, we plot the calculated mode Grüneisen parameters of these materials in Fig. 5e . The TO modes in lead chalcogenides and SnTe have remarkably large mode Grüneisen parameters. Bi 2 Te 3 , Bi and Sb also have increasing Grüneisen parameters as the zone center is approached, but the magnitude is not as large as in IV–VI materials. The strong anharmonic TO modes in IV–VI materials lead to their low lattice thermal conductivities and this was predicted and experimentally observed [30] , [31] , [32] , [33] , [34] . In Fig. 6 , we show detailed phonon transport characteristics in several III–V and IV–VI materials, calculated from the density functional theory. We calculate phonon transport of SnTe and InSb in addition to PbTe, PbSe and GaAs from literature [33] , [35] . It is interesting to directly compare SnTe and InSb as these materials are close to each other in the periodic table, and therefore they have a similar Debye temperature and mass ratio. The thermal conductivity calculation of InSb using first-principles was recently reported [36] . The calculated and experimental thermal conductivity values in Fig. 6a show large contrast between III–V and IV–VI materials. We further contrast the two different material groups by analysing the phonon mean-free path and phonon lifetime. For the phonon mean-free path, we present accumulated thermal conductivity as a function of the phonon mean-free path at 300 K, defined as , where Λ , q , s and χ represent the phonon mean-free path, wavevector, polarization and a step function, respectively [37] , [38] . The accumulated thermal conductivity function shows the mean-free path ranges of phonon modes that significantly contribute to thermal conductivity. From Fig. 6b,c , it is clearly seen that the IV–VI materials exhibit much shorter mean-free path ranges and phonon lifetime compared with the III–V materials. The significant effect of soft TO mode on lattice thermal conductivity is also substantiated by the comparison between PbTe and Bi. The thermal conductivity of PbTe is smaller than that of Bi by a factor of two, although atomic mass of PbTe is less than that of Bi (refs 39 , 40 ) (see Supplementary Note 6 for details). 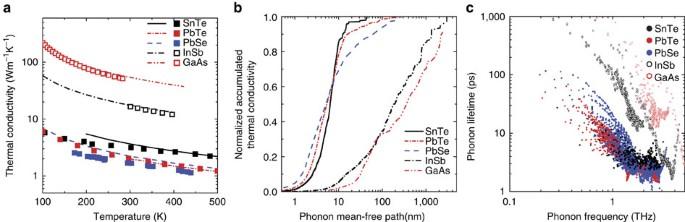Figure 6: Analysis of phonon transport in IV–VI and III–V materials by first-principles calculation. (a) Calculated and experimental lattice thermal conductivities. Lines and squares are results by experiments and calculations, respectively. (b,c) Phonon mean-free path distributions and phonon lifetime, showing significant three-phonon scattering in IV–VI materials. The accumulated thermal conductivity is normalized by the thermal conductivity value of each material. The data in (b,c) are for 300 K case. The experimental thermal conductivity data in (a) are from refs7,8,39,52and the calculation results for PbTe, PbSe and GaAs are from refs33,35. Figure 6: Analysis of phonon transport in IV–VI and III–V materials by first-principles calculation. ( a ) Calculated and experimental lattice thermal conductivities. Lines and squares are results by experiments and calculations, respectively. ( b , c ) Phonon mean-free path distributions and phonon lifetime, showing significant three-phonon scattering in IV–VI materials. The accumulated thermal conductivity is normalized by the thermal conductivity value of each material. The data in ( b , c ) are for 300 K case. The experimental thermal conductivity data in ( a ) are from refs 7 , 8 , 39 , 52 and the calculation results for PbTe, PbSe and GaAs are from refs 33 , 35 . Full size image In addition to the phonon anharmonicity, the phonon lifetimes also depend on the three-phonon scattering phase space available that meets energy and momentum conservation requirements. The difference in the volume of the scattering phase space explains the second difference between III–V and IV–VI materials in Fig. 1 (that is, the thermal conductivity difference between III–V and IV–VI materials is much increased when the mass difference between the two atoms is large). To compare IV–VI and III–V materials, we plot the inverse of the three-phonon scattering phase-space volume of these materials in Fig. 7a . Assuming constant phonon anharmonicity, the inverse of the three-phonon scattering phase-space volume relates linearly to phonon lifetime and hence thermal conductivity. Since the scattering phase space is inversely proportional to the frequency scale, the integrated volume of the phase space of each material is normalized by the inverse of maximum optical phonon frequency to compare many materials with different phonon frequency scale. The phase-space volume for III–V we calculated is similar to the previously reported data using a bond charge model [41] . From Fig. 7a , we can see that III–V materials with dissimilar atomic masses such as AlSb and InP have much smaller phase spaces than other III–V materials. This is a common behaviour for many materials that have large atomic mass differences [42] . The large mass difference causes a large gap to appear between the acoustic and optical phonon bands as shown in Fig. 7b . With such a large gap, low-frequency acoustic phonons cannot couple to optical phonons and thus have fewer chances to be scattered. Only high-frequency acoustic phonons, which are localized in a small region of reciprocal space, can be coupled with optical phonons. As the mass ratio is reduced from unity, the acoustic optical phonon gap becomes larger and the scattering phase space is further reduced, leading to longer lifetimes and larger thermal conductivities. As can be seen from Fig. 7c , the phase space in AlSb is mostly due to (a,a,a) and the phase spaces of (a,a,o) and (a,o,o) are significantly suppressed. (‘a’ and ‘o’ in (a,a,o) indicate acoustic and optical phonons in the three-phonon process.) 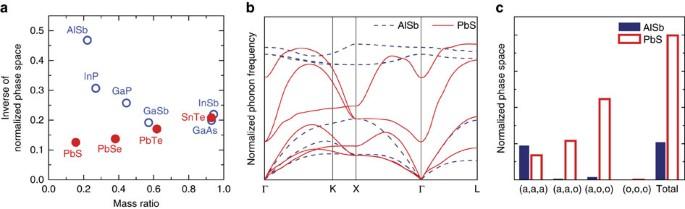Figure 7: Phase-space volume for three-phonon scattering. (a) Phase-space volumes for three-phonon scattering of IV–VI and III–V, showing the large scattering phase space of PbSe and PbS. (b) Comparison of the phonon dispersion of PbS and AlSb, showing significantly dispersed optical phonons of PbS. (c) Contribution of each scattering channel to total scattering phase-space volume. The scattering phase space and phonon dispersion data are normalized by the inverse of the largest optical phonon frequency of each material for comparison. Figure 7: Phase-space volume for three-phonon scattering. ( a ) Phase-space volumes for three-phonon scattering of IV–VI and III–V, showing the large scattering phase space of PbSe and PbS. ( b ) Comparison of the phonon dispersion of PbS and AlSb, showing significantly dispersed optical phonons of PbS. ( c ) Contribution of each scattering channel to total scattering phase-space volume. The scattering phase space and phonon dispersion data are normalized by the inverse of the largest optical phonon frequency of each material for comparison. Full size image The three-phonon scattering pathway in IV–VI materials is much different from that of III–V materials since the (a,o,o) channel significantly contributes to the total phase-space volume in IV–VI materials. The difference in the scattering pathway between III–V and IV–VI materials can be easily observed in Fig. 7a ; the phase-space volume of IV–VI materials increases slightly as the mass ratio decreases, an opposite trend to the case of III–V materials. The reason for this opposite trend is that the (a,o,o) channel is a large contributor to total phase-space volume in IV–VI materials, and this scattering channel is affected by the overlap between acoustic and optical bands (see Supplementary Note 7 for detailed discussions). The large phase-space volume of the (a,o,o) process can be explained with the wide spectrum of optical modes. The bandwidth of the optical phonons is comparable to the bandwidth of the acoustic phonons. As a result, most acoustic phonons from very low frequencies to high frequencies can participate in the (a,o,o) process, widening the (a,o,o) channel in IV–VI materials. In particular, the (a,o,o) process in PbS contribute more than half of the total phase space. In addition, the (a,a,o) channel also considerably contributes to total phase-space volume in the case of PbS, while it is almost negligible in AlSb. This is owing to the reduced phonon band gap by soft TO mode; with the reduced phonon band gap, most acoustic phonons, regardless of frequency, can be scattered by a TO mode contributing to the (a,a,o) process, while only high-frequency acoustic phonons can participate in the (a,a,o) process when the gap is large. The large (a,o,o) and (a,a,o) scattering phase space of PbSe and PbS suggests that acoustic phonons are effectively scattered by optical phonons, exhibiting low thermal conductivity values despite the small mass ratio as shown in Fig. 1 . We have presented the effects of resonant bonding on lattice dynamics characteristics and thermal conductivity. We revealed that materials with resonant bonding (lead chalcogenides, SnTe, Bi 2 Te 3 , Bi and Sb) commonly have long-ranged interactions along the 〈100〉 direction in rocksalt structure. This long-ranged interaction is significant in IV–VI materials owing to the strong resonant bonding, and results in the near-ferroelectric instability in these materials. However, the long-ranged interaction is less significant with increasing distortion of the crystal structures as in Bi. The near-ferroelectric behaviour caused by the resonant bonding reduces the lattice thermal conductivity through two mechanisms: strong anharmonic scattering and a large scattering phase-space volume, both due to softened optical phonons, resulting in the lower thermal conductivities of IV–VI materials compared with III–V compounds. Thus, the low thermal conductivities of these materials are traced back to their crystal structure and electronic occupation (the resonant nature of the bonding). Our findings have significant implications for designing better thermoelectric and phase-change materials. The fundamental understanding of lattice dynamics from chemical bonding points to the potential to search for good thermoelectric materials through the resonant bonding picture. Also, we showed a deep connection among ferroelectric, thermoelectric and phase-change materials. These insights help researchers to explore better thermoelectric and phase-change materials. Lattice dynamics calculation We used the density functional perturbation theory to calculate harmonic lattice dynamics properties of the materials [43] , [44] . We checked that results are well converged with respect to many parameters such as cutoff energy of plane wave basis and reciprocal space sampling size ( k - and q - grid). We provide detailed calculation conditions for each material in Supplementary Table 1 . Since the long-ranged interaction is significant in the resonant bonding materials, we used a relatively fine q -grid to capture the long-ranged interaction. Also, for heavy elements such as Bi, Pb, Te, Sb and Se, spin-orbit interaction is included in the calculation. After calculating IFC tensors, we normalize the trace of the IFC tensor to compare many materials with different crystal structures and different strengths of bonding ( Supplementary Note 2 for details). To calculate mode Grüneisen parameter, we calculated phonon frequencies for two cases: equilibrium volume and expanded volume by 1%. Then, we took differences in phonon frequencies of two cases and calculate Grüneisen parameter by its definition, γ =− Vdω / ωdV . The calculations were performed with the QUANTUM ESPRESSO for lead chalcogenides and SnTe and the ABINIT package for other materials [45] , [46] . Electron density distribution To confirm that electron polarization is long ranged in PbTe, but short ranged in NaCl, we calculated electron density distributions in PbTe and NaCl using density functional theory for two different cases: without any displacement and with small displacement of one atom. We displaced a Pb atom and a Na atom for PbTe and NaCl, respectively. The displacement is 2% of the fourth-nearest neighbour distance in − x direction in Fig. 4 . Since a periodic boundary condition is used in the electron distribution calculation, there is an effect from the periodic images of the displaced atom. Therefore, we calculated large enough supercells (24 atoms) to minimize this effect. Other calculation conditions are same as the phonon calculation conditions in Supplementary Table 1 . After calculating electron density of two cases, we took the finite difference of two cases to calculate change in electron density distribution by the displacement. Phase-space volume for three-phonon scattering The phase-space integral for three-phonon scattering is the volume satisfying energy and momentum conservation in the three-phonon process. Therefore, it can be defined as [41] where j , j ′ and j ′′ represent phonon branches. The two δ -functions are for energy conservation of coalescent and decay processes. The superscripts, q + q ′− G and q − q ′− G denote momentum conservation. The factor of half in front of the second term (decay process) is to prevent counting twice when summing up all the possible scattering pathways. For the integration of the δ -functions, we used a q -grid of 20 × 20 × 20 and confirmed the convergence of phase space with respect to the q -grid size. As seen in the expression for phase-space volume above, phase-space volume is integration of δ -functions of phonon frequencies. Therefore, the phase-space volume is inversely proportional to phonon frequency scale. To compare many materials with different phonon frequency scales, we normalized the phase-space volume by the inverse of maximum optical phonon frequency. To validate the phonon dispersion used in the phase-space volume calculation, we present calculated phonon dispersions compared with the experimental data in Supplementary Figs 15 and 16 . Lattice thermal conductivity from first-principles We used the density functional theory to calculate lattice thermal conductivity of InSb and SnTe. Here we briefly present the method we used and more details are available in other literature [47] . We calculate second-order force constants using the density functional perturbation theory and the calculation conditions for the force constants are shown in Supplementary Table 1 . The calculated second-order force constants were validated by comparing the calculated phonon dispersion to the experimental data in Supplementary Figs 15 and 16 . For third-order force constants, we calculate forces on atoms in large enough supercells (4 × 4 × 4 supercells, 128 atoms) with various atomic displacements. The set of third-order force constants, minimally reduced by symmetry considerations, is then fitted to the calculated force-displacement data with enforcing translational and rotational invariances [48] . We considered up to second-nearest neighbours and fifth-nearest neighbours for the third-order force constants of InSb and SnTe, respectively. The thermal expansion coefficients were calculated using the second- and third-order force constants, showing reasonable agreement with the experimental values ( Supplementary Note 8 ). The calculated second- and third-order force constants gives the rate of three-phonon scatterings via Fermi’s golden rule and also other properties such as phonon frequency and group velocity. Then, with all these information, the lattice thermal conductivity was calculated by solving Boltzmann equation under relaxation time approximation. How to cite this article: Lee, S. et al . Resonant bonding leads to low lattice thermal conductivity. Nat. Commun. 5:3525 doi: 10.1038/ncomms4525 (2014).